Mutational landscape of intrahepatic cholangiocarcinoma Intrahepatic cholangiocarcinoma (ICC) is a fatal primary liver cancer (PLC) that affects 5–10% of all PLCs. Here we sequence tumour and matching control sample pairs of a large cohort of 103 ICC patients in China, resulting in the identification of an ICC-specific somatic mutational signature that is associated with liver inflammation, fibrosis and cirrhosis. We further uncover 25 significantly mutated genes including eight potential driver genes ( TP53 , KRAS , IDH1 , PTEN , ARID1A , EPPK1 , ECE2 and FYN ). We find that TP53 -defective ICC patients are more likely to be HBsAg-seropositive, whereas mutations in the oncogene KRAS are nearly exclusively found in HBsAg-seronegative ICC patients. Three pathways (Ras/phosphatidylinositol-4,5-bisphosphate 3-kinase signalling, p53/cell cycle signalling and transforming growth factor-β/Smad signalling), genes important for epigenetic regulation and oxidative phosphorylation are substantially affected in ICC. We reveal mutations in this study that may be valuable for designing further studies, better diagnosis and effective therapies. The intrahepatic cholangiocarcinoma (ICC, also abbreviated as IHCC or IH-CCA) is a fatal primary liver cancer (PLC) arising from the epithelial lining of the peripheral intrahepatic bile duct epithelium [1] . Globally, PLC is the fifth most common cancer with about 600,000 annual deaths [2] . ICCs account for 5–10% of all PLCs in western countries [3] , [4] , compared with the hepatocellular carcinoma (HCC) that account for about 90% of all PLCs [5] . Despite the relative low incidence of ICC, it deserves urgent attention because the worldwide incidence of ICC has been increasing steadily and substantially over the last 30 years, from 0.32 to 0.85 per 100,000 people, an 165% increase [6] . In Asian countries, the incidence is alarmingly much higher than the worldwide incidence [7] . For example, ICC affects 96 per 100,000 people in Thailand, an incidence 100-fold higher than the worldwide average [8] . In addition to the increasing incidence, the prognosis of ICC is devastating and the mortality rate is high [1] , because patients diagnosed with ICC are usually at advanced stages because of lack of appropriate markers for early conclusive diagnosis [9] . Currently, surgical removal is considered the only choice of treatment of ICC [1] . However, the surgery outcome is grim, with the median survival after hepatic resection 12.2 months, although it is better than the median survival after conservative therapy (1.8 months) [10] . Thus, in order to achieve earlier and more accurate diagnosis for better therapeutic outcome, knowledge of the somatic mutations that trigger the tumorigenesis of ICC is an essential first step. In recent years, genomic research on PLCs has been overwhelmingly focusing on HCC. Many large-scale genome sequencing projects have been executed to identify how somatic mutations [11] , [12] , [13] , [14] , [15] , [16] , [17] , [18] and hepatitis B virus (HBV) integration [19] , [20] , [21] affect HCC patients. In contrast, large-scale genome sequencing projects targeting the ICC cancer genomes just started to catch up. A recent project searched for genome-wide somatic mutations in a small cohort of eight patients with cholangiocarcinoma associated with liver fluke infection [22] . Very recently, two sequencing projects reported novel mutations in relatively larger cohorts of ICC patients [23] , [24] , revealing two striking features of ICC. First, these studies revealed high genetic heterogeneity of ICC. For example, in a cohort of 32 ICC patients in the discovery screen and an additional 32 ICC patients in the prevalence screen, no single gene was mutated in >25% of the ICC tumours screened [24] . Second, these studies revealed striking uniqueness in mutation prevalence of key genes between different cohorts of ICC patients, suggesting important contribution of genetic differences of the ICC patients and different risk factors to the mutational landscape. For example, the three frequently mutated genes BAP1 , ARID1A and PBRM1 found in a more recent project [24] were completely missing in the earlier study [22] . In addition, ICC patients with liver fluke infection in Thailand showed dramatic differences in mutated genes from those without infection in Singapore [23] . For example, 7.4% of non- O. viverrini ICC patients in Singapore carry mutations in TP53 , compared with 45.2% of O. viverrini ICC patients in Thailand. Therefore, to better understand the tumorigenesis of ICC, genome sequencing and analysis of additional cohorts of ICC patients from different environments (thus different pathological factors) and with different genetic backgrounds are needed. In particular, the size of new ICC discovery cohorts need to be much larger (compared with 8 (ref. 22 ), 15 (ref. 23 ) and 32 (ref. 24 ) patients in the three previous studies) to ensure better representation of mutations in different ICC patients, and the new ICC patient cohorts should represent different genetic background and risk factors. This project represents the first project that aims to identify somatic mutations in a large cohort of ICC patients in China through exome sequencing. Through sequencing the exomes of tumour and matching control sample pairs of a large cohort of 103 ICC patients in China, we identify 9,713 somatic synonymous and non-synonymous mutations, which affect 3,637 genes. We find that 25 genes are significantly mutated genes, 8 of which ( TP53 , KRAS , IDH1 , PTEN , ARID1A , EPPK1, ECE2 and FYN ) show significant positive selection, suggesting that these genes are likely driver genes. Mutation spectrum in ICC genomes We analysed a cohort of 103 ICC patients who underwent surgical dissection for ICC in the Eastern Hepatobiliary Surgery Hospital of the Second Military Medical University (Shanghai, China) between March 2009 and March 2011 ( Supplementary Note 1 and Supplementary Data 1 ). We generated 1,245 and 1,157 Gb exome DNA sequence data from the tumour and matching control samples ( Supplementary Data 2 ). The average coverage of the coding exons in the tumour and the control samples are 80- and 76-folds, respectively. On average, 92% of the coding regions of both the tumour and the control samples have 15-fold coverage or higher. We have identified 9,713 somatic synonymous and non-synonymous mutations (including single-nucleotide mutations and small insertions and deletions, or indels; Supplementary Data 3 ), averaging 94.3 somatic mutations per ICC patient. The numbers of somatic mutations vary dramatically, ranging from 16 (patient p89) to 1,333 (patient p119). The high density of mutations (39.3/Mb) in patient p119 is in the same range as those other types of cancer patients with defective DNA mismatch repair mechanism mutations in DNA-repairing mechanisms [25] . Indeed, somatic mutations are found in three genes ( PARP4 , DDB1 and SSBP1 ) that can play critical roles in DNA repairing. This patient is thus excluded from further analysis. We used somatic mutations found from 102 ICC patients to identify statistically significant mutations. For follow-up survival analysis of ICC patients harbouring different mutated genes, we focused on 101 patients (excluding p119 mentioned above and patient p97 who died of unrelated cerebral haemorrhage). 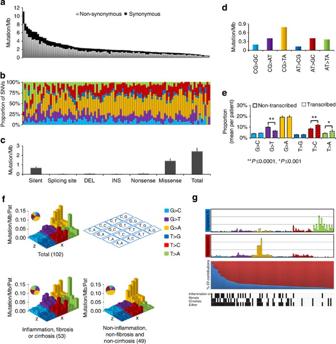Figure 1: Mutation spectrum revealed by whole-exome sequencing in 102 ICC patients. (a) Somatic mutation density (mutations per Mb) in 102 ICC patients. Non-synonymous and synonymous are separated into two categories. (b) Proportion of six types of single-nucleotide substitutions in 102 patients sorted by the order as Fig. 1a. Different types of single nucleotide variants (SNVs) are consistently coloured in this figure. (c) Rate of different types of somatic mutations. (d) Mean of six types of SNVs and indels in 102 ICC patients. (e) Types of SNVs on transcribed strand and non-transcribed strand.P-value is estimated by paired Student’st-test. (f) Triple-nucleotide mutation context. Six types of point mutations are reflected by six colour-coded blocks. Each block has 16 columns, indicating different flanking nucleotides of mutation sites. The ‘Pie chart’ shows the proportion of each type of point mutations. (g) Mutation signatures. The upper panel shows two mutation signatures predicted by the programme EMu. The lower panel shows the percentage of the contributions of two pathological features in each ICC patient, correlating with liver inflammation or fibrosis (upper), cirrhosis (middle) and liver inflammation, fibrosis or cirrhosis (lower). The density of somatic mutations in the 102 ICC patients (2.4/Mb; Table 1 ) is similar to other types of solid tumours [25] . Table 1 Summary of exome sequencing results of tumour-control pairs from 102 ICC patients. Full size table We have selected all 1,103 predicted somatic mutations found in genes mutated in three or more ICC patients for validation by Sanger sequencing. Among these, we obtained unambiguous results for 1,032, of which 923 (89.4%) are in concordance with our predictions ( Supplementary Data 4 ), indicating high quality of mutation detection. Only validated mutations are used in further functional analysis. Among all mutations, C:G>T:A transition is the most frequent change ( Fig. 1b,d,e ), a feature shared by HCCs [11] , [12] , [13] , [14] and cholangiocarcinomas (CCAs) [22] , and essentially all tumour types that have been sequenced [25] . In particular, the C>T transition observed in ICC patients in our study is found to be more enriched in CpG sites (yellow bars in Fig. 1f ), as also observed in other cancers [25] and in cholangiocarcinomas (CCAs). [22] . Notably, three types of point mutations found in ICC show significant strand bias: G>T substitution is significantly more frequent in the non-transcribed strand, whereas the T>C and T>A substitutions are significantly more frequent in the transcribed strand ( Fig. 1e ). Strand-biased G>T mutation patterns were also observed in a cohort of HCC patients from France [13] , suggesting a similar mechanism underlying the formation of such bias in these two types of PLCs. In addition to the elevated C>T substitutions in the CpG sites, we also uncovered high rates of the CTG>CAG and CAG>CTG changes (the tallest green bar in Fig. 1f ). This feature has not been described in any of the 27 tumour genomes analysed recently [26] , nor has it been observed in the liver fluke-associated CCA genomes [22] . These two mutational signatures were also discovered in an unbiased exploration using EMu [27] as two unique mutation signatures ( Fig. 1g ): Signature A (green bars) and B (yellow bars). Figure 1: Mutation spectrum revealed by whole-exome sequencing in 102 ICC patients. ( a ) Somatic mutation density (mutations per Mb) in 102 ICC patients. Non-synonymous and synonymous are separated into two categories. ( b ) Proportion of six types of single-nucleotide substitutions in 102 patients sorted by the order as Fig. 1a. Different types of single nucleotide variants (SNVs) are consistently coloured in this figure. ( c ) Rate of different types of somatic mutations. ( d ) Mean of six types of SNVs and indels in 102 ICC patients. ( e ) Types of SNVs on transcribed strand and non-transcribed strand. P -value is estimated by paired Student’s t -test. ( f ) Triple-nucleotide mutation context. Six types of point mutations are reflected by six colour-coded blocks. Each block has 16 columns, indicating different flanking nucleotides of mutation sites. The ‘Pie chart’ shows the proportion of each type of point mutations. ( g ) Mutation signatures. The upper panel shows two mutation signatures predicted by the programme EMu. The lower panel shows the percentage of the contributions of two pathological features in each ICC patient, correlating with liver inflammation or fibrosis (upper), cirrhosis (middle) and liver inflammation, fibrosis or cirrhosis (lower). Full size image Although the C:G>A:T mutation is common in most cancer types, the CTG>CAG and CAG>CTG mutations are unique to ICC. The cause of this unique mutation feature is unknown. To explore the cause of this unique mutation feature, we have traced and examined the aetiological factors that may play a role in mutagenesis. Among the aetiological factors including alcohol consumption, smoking, fatty liver, HBV infection, hypertension, the unique mutation signature is only positively associated with liver inflammation, fibrosis and cirrhosis as revealed in pathological examination of the liver condition ( Fig. 1f ). Patients with liver inflammation or fibrosis alone ( P =0.011, Kolmogorov–Smirnov test) or cirrhosis alone ( P =0.001, Kolmogorov–Smirnov test) are significantly enriched with A:T>T:A mutations (all green bars in Fig. 1f ). Patients with liver inflammation, fibrosis or cirrhosis are even more significantly enriched with A:T>T:A mutations ( P <0.001, Kolmogorov–Smirnov test). Furthermore, patients with liver inflammation or fibrosis alone ( P =0.043, Kolmogorov–Smirnov test) or cirrhosis alone ( P =0.025, Kolmogorov–Smirnov test) are significantly enriched with the CTG>CAG and CAG>CTG mutations (that is, the tallest green bar in Fig. 1g ). Patients with liver inflammation, fibrosis or cirrhosis are even more significantly enriched with the CTG>CAG and CAG>CTG mutations ( P <0.001, Kolmogorov–Smirnov test). Our results suggest that mutagens that caused liver inflammation, fibrosis or cirrhosis may be associated with the A:T>T:A mutations. As shown in Fig. 1g , some patients of our ICC cohort have higher content of Signature A mutations, whereas others have higher content of Signature B mutations. ICC patients with higher Signature A content are strongly correlated with inflammation, fibrosis or cirrhosis, whereas ICC patients with more Signature B are less likely to have these aetiological features. Significantly mutated genes Among the 3,637 genes that are affected by somatic mutations (excluding somatic mutations that are also found in dbSNP and the 1000 Genome Project) in the 102 ICC patients ( Table 1 ), most are mutated only in single ICC patients. 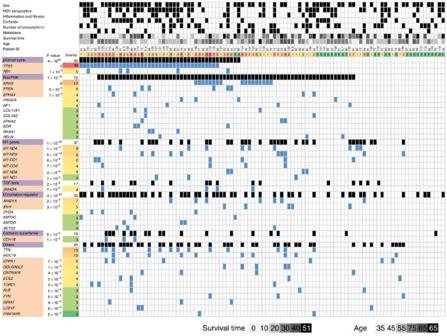Figure 2: Significantly mutated genes and pathways in ICC and their association with major clinical features. The major clinical features, survival time and age are listed above patient ID, whereas the mutations for each patient in these significantly mutated genes are displayed underneath the patient ID. In the ‘Sex’ row, black cells represent male, whereas white cells represent female. In the next five rows (‘HBV seropositive’, ‘Inflammation and fibrosis’, ‘Cirrhosis’, ‘Number of tumours’ and ‘Metastasis’), black cells represents patients positive for the corresponding clinical feature, whereas white cells represents patients negative for the corresponding clinical feature. In the ‘Survival time’ and ‘Age’ rows, the intensity of the cells represent years (as illustrated at the bottom of the figure). To the left of mutational panel, significantly mutated genes (highlighted in light brown) are reported and categorized in major common altered pathway (highlighted in purple). For each patient, potentially altered pathways (black cells) are affected by non-synonymous somatic mutations (blue cells). In this figure, only validated mutations (mutations in genes significantly mutated or mutated in more than two patients) are shown. The ‘Events’ values in horizontal row show numbers of significantly mutated genes for every patient, whereas those in vertical column reflect numbers of mutated patients for each pathway or gene. The significance levelP-value is calculated by Genome-MuSiC. Applying Genome-MuSiC [28] , we found a set of 25 significantly mutated genes ( Table 2 ; Fig. 2 ; Supplementary Data 5 and 6 ). To estimate selection pressure on these 25 significantly mutated genes in the tumorigenesis of ICC, we have further determined the significance of observed non-synonymous/synonymous ratios of these 25 significantly mutated genes over expected non-synonymous/synonymous ratios using an exact Monte Carlo test [25] . Among these 25 genes, 8 genes TP53 ( P =0.00001), KRAS ( P =0.004), IDH1 ( P =0.00019), PTEN ( P =0.0078), ARID1A ( P =0.00449), EPPK1 ( P =0.00486), ECE2 ( P =0.0357) and FYN ( P =0.00258) showed significant positive selection, suggesting that these genes are likely driver genes. However, recent studies have demonstrated that genes with synonymous mutations could also be driver genes and play important role in tumorigenesis [29] , [30] . Therefore, other genes in Table 2 could be potential driver genes as well. Among these genes, two genes TP53 and ARID1A are also frequently mutated in HCC patients [12] , [13] , [14] , [15] , [17] , [18] , suggesting that these two types of PLCs may have both unique and shared molecular mechanisms in tumorigenesis. TP53 is mutated in 39 (38.2%) of this cohort of ICC patients, a frequency within the range of frequencies reported in some previous studies targeting TP53 in ICCs, but is substantially higher than many frequencies reported previously. For example, this frequency is much higher than that (6%) reported in the cohort of 32 ICC patients treated at various hospitals in the United States of America [24] , that (9.8%) reported in the cohort of 41 ICC patients from Singapore [23] and that (8.9%) reported in the cohort of 45 ICC patients from Romania [23] . These patients (who are from Singapore and Romania) and patients studied here do not have liver fluke infection, suggesting that factors other than liver fluke infection contributed to the differences in mutation prevalence. On the contrary, the frequency is similar to that (39.8%) reported in the cohort of 108 ICC patients who are infected by liver fluke. Thus, the differences in mutation prevalence of TP53 in different cohorts of ICC patients from different countries cannot be simply explained by whether the patients are infected by liver fluke. Instead, it suggests a combination of genetic background and exposure to risk factors has contributed to the mutation prevalence observed in ICC patients in different countries. Table 2 Significantly mutated genes in the 102 ICC patients. Full size table Figure 2: Significantly mutated genes and pathways in ICC and their association with major clinical features. The major clinical features, survival time and age are listed above patient ID, whereas the mutations for each patient in these significantly mutated genes are displayed underneath the patient ID. In the ‘Sex’ row, black cells represent male, whereas white cells represent female. In the next five rows (‘HBV seropositive’, ‘Inflammation and fibrosis’, ‘Cirrhosis’, ‘Number of tumours’ and ‘Metastasis’), black cells represents patients positive for the corresponding clinical feature, whereas white cells represents patients negative for the corresponding clinical feature. In the ‘Survival time’ and ‘Age’ rows, the intensity of the cells represent years (as illustrated at the bottom of the figure). To the left of mutational panel, significantly mutated genes (highlighted in light brown) are reported and categorized in major common altered pathway (highlighted in purple). For each patient, potentially altered pathways (black cells) are affected by non-synonymous somatic mutations (blue cells). In this figure, only validated mutations (mutations in genes significantly mutated or mutated in more than two patients) are shown. The ‘Events’ values in horizontal row show numbers of significantly mutated genes for every patient, whereas those in vertical column reflect numbers of mutated patients for each pathway or gene. The significance level P -value is calculated by Genome-MuSiC. Full size image Among the 39 mutations identified in this study, although most are truncating mutations ( Fig. 3a ), 10 occur at the codon 249 (R249S). This R249S mutation in TP53 has been frequently reported in HCC patients confers a growth advantage for HCC cells [31] but has never been reported in ICC patients in previous studies. The R249S mutation is a demonstrated signature of aflatoxin-induced mutation [32] , suggesting that ICC patients with this mutation may have been exposed to aflatoxin, which is one type of mycotoxins produced by the common fungi Aspergillus flavus and Aspergillus parasiticus and has been classified as a group I carcinogen in humans by IARC [33] . Furthermore, this observation may suggest that aflatoxin may play an important role in the pathogenesis of this cohort of ICC patients in China as a risk factor for ICC, which is consistent to the widespread aflatoxin contamination in cereals, oils and foodstuffs in Southern China [34] , where most ICC patients studied in this project lived ( Supplementary Note 1 ). 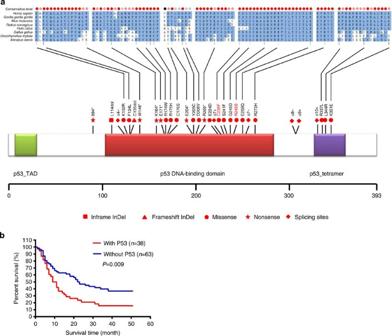Figure 3: Mutations inTP53and their impact on ICC patient survival. (a) Sites of amino-acid changes in p53 due to mutations inTP53. Conservation of these sites was evaluated by the multiple sequence alignment ofTP53orthologues in man (Homo sapiens), gorilla (Gorilla gorilla gorilla), mouse (Mus musculus), rat (Rattus norvegicus), cat (Felis catus), chicken (Gallus gallus), rainbow trout (Oncorhynchus mykiss) and frog (Xenopus leavis). (b) Comparison of survival of ICC patients withTP53mutations (With P53) and withoutTP53mutations (Without P53). Survival analysis was done using SPSS. Figure 3: Mutations in TP53 and their impact on ICC patient survival. ( a ) Sites of amino-acid changes in p53 due to mutations in TP53 . Conservation of these sites was evaluated by the multiple sequence alignment of TP53 orthologues in man ( Homo sapiens ), gorilla ( Gorilla gorilla gorilla ), mouse ( Mus musculus ), rat ( Rattus norvegicus ), cat ( Felis catus ), chicken ( Gallus gallus ), rainbow trout ( Oncorhynchus mykiss ) and frog ( Xenopus leavis ). ( b ) Comparison of survival of ICC patients with TP53 mutations (With P53) and without TP53 mutations (Without P53). Survival analysis was done using SPSS. Full size image In general, mutations in TP53 are associated with worse survival of our cohort of 101 ICC patients ( P =0.009; Fig. 3b ). Our ICC patients with somatic mutations in TP53 are more likely to be HBsAg-seropositive ( P =0.021), suggesting that p53-mediated pathway may contribute to the tumorigenesis of HBV-infected HCC and ICC patients, supporting a recent hypothesis that HBV-infected ICC and HCC may hold common disease process for carcinogenesis [35] . Although ICC patients with somatic mutations in TP53 are positively associated with HBsAg, not all HBsAg-seropositive patients have somatic mutations in TP53 . Survival analysis suggested that HBsAg-seropositive patients without somatic mutations in TP53 have better prognosis compared those with somatic mutations in this gene ( P =0.014). Thus, the combination of mutations in TP53 and the presence of HBsAg can be used as indicators of prognosis of ICC patients. A significantly mutated gene in our ICC patients that has rarely been found to be mutated in HCC is v-Ki- ras2 Kirsten rat sarcoma viral oncogene homologue ( KRAS ). KRAS is mutated in 16.7% in our cohort of 102 ICC patients and is the second most common significantly mutated gene ( Fig. 2 ). Similar mutation rate of KRAS (16%) was reported for the CCA patients from Thailand [22] . The percentage of patients who have mutations in KRAS is remarkably similar between these two cohorts of patients, despite that the 54 CCA patients are associated with liver fluke, whereas none of the 102 ICC patients are associated with this parasite, suggesting that factors other than liver fluke infection contributes to the incidences of KRAS mutation. Our cohort of ICC patients also shows mutation spectral difference from these liver fluke-associated CCA in many genes including GNAS , which is mutated in 9.2% of the liver fluke-associated CCA patients [22] , but only in a single ICC patient (1.0%) in this study. Previous targeted sequencing efforts have come to markedly different mutation rates for KRAS in patients from different Asian and European countries, which may be associated with the aetiologies specific to patients from different locations. In sharp contrast, KRAS was not identified as significantly mutated gene in any HCC cancer genome sequencing projects [12] , [13] , [14] , [15] , [16] , [17] , [18] , underscoring the uniqueness between these two types of PLCs. Among 17 KRAS mutations discovered in our study, all mutations occur exclusively at codon 12, causing G->D (seven), G->V (six), G->A (two) and G->C (two) changes in the protein ( Supplementary Data 3 ). ICC patients with mutations in KRAS show worse survival compared with those without such mutations ( P =0.044; Fig. 4a ). Mutations in KRAS are frequently found in HBsAg-seronegative ( P =0.001), consistent with the overall worse survival of HBsAg-seronegative ICC patients [36] . 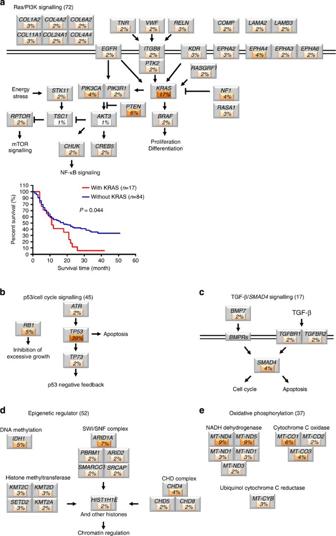Figure 4: Significantly altered pathways in ICC. Mutation frequencies are expressed as the percentage under the gene names. In this figure, in most cases, only genes mutated more than one patient are shown in the pathway. (a) Genes mutated in the Ras/PI3K signalling pathway, comparison of survival of ICC patients withKRASmutations (withKRAS) and withoutKRASmutations (withoutKRAS); (b) p53/cell cycle signalling pathway; (c) TGF-β/SMAD signalling pathway; (d) epigenetic regulators; (e) Oxidative phosphorylation. Survival analysis was done using SPSS. The colour intensity of the boxes represents the number of ICC patients who carry mutations in the gene. Figure 4: Significantly altered pathways in ICC. Mutation frequencies are expressed as the percentage under the gene names. In this figure, in most cases, only genes mutated more than one patient are shown in the pathway. ( a ) Genes mutated in the Ras/PI3K signalling pathway, comparison of survival of ICC patients with KRAS mutations (with KRAS ) and without KRAS mutations (without KRAS ); ( b ) p53/cell cycle signalling pathway; ( c ) TGF-β/SMAD signalling pathway; ( d ) epigenetic regulators; ( e ) Oxidative phosphorylation. Survival analysis was done using SPSS. The colour intensity of the boxes represents the number of ICC patients who carry mutations in the gene. Full size image In addition to frequently mutated genes TP53 and KRAS , our exome sequencing effort also identified mutations in SMAD4 (3.9%), RB1 (4.9%), IDH1 (4.9%) and ARID1A (6.9%) that have been found to be mutated in ICC in previous studies [22] , [23] , [24] , [37] , [38] , [39] , [40] , [41] . Of importance, we have uncovered a set of significantly mutated genes that have not previously found to be associated with ICC: PTEN , GOLGA6L2 , EPHA4 , EPPK1 , CDH18 , ALB , FAM182B, ECE2 , TDRD1 , GRIA1 , CNTNAP5 and FYN . Evidence from previous publications suggests that some likely play important role in ICC. For example, although mutations in PTEN , which encodes a Ras/phosphatidylinositol-4,5-bisphosphate 3-kinase (PI3K) signalling pathway component phosphatase and tensin homologue (PTEN) [42] , have not previously been found in human ICC patients, mice with liver-specific disruption of both PTEN and SMAD4 , which encodes a common mediator of the transforming growth factor (TGF)-β/Smad4 signalling pathway [43] , specifically developed ICC, whereas disruption of SMAD4 alone did not lead to the development of ICC [44] . This study suggests a unique role of mutations in PTEN in the tumorigenesis of ICC. Similarly, although mutations in ARID1A have not been found in a previous study on a cohort of 54 ICC patients with liver fluke infection, mutations in this gene have been found in two recent studies with larger sample sizes [23] , [24] , suggesting the importance of obtaining larger cohorts of ICC patients in mutation discovery studies. They have also been reported in multiple HCC cancer genomics [12] , [13] , [14] . Functional analysis of the role of ARID1A by suppression its expression using RNA interference indicated that loss-of-function of ARID1A promoted proliferation, migration and invasion [14] . The functional contribution of most of the significantly mutated genes is still unknown, thus providing a rich resource for further research on the mechanisms underlying the tumorigenesis of ICC. Signalling pathways affected in ICC Many mutated genes, including ones mutated only in small subsets of ICC patients, constitute members of important signalling pathways. Thus, we analysed the impact of mutations in these genes in the context of signalling pathways, which may help us understand the similarity and differences between the pathogenesis of ICC and HCC and the uniqueness of mutations in ICC. Based on annotation at Kyoto Encyclopedia for Genes and Genomes (KEGG) databases [45] , three major signalling pathways Ras/PI3K, p53/cell cycle and TGF-β/SMAD4 are substantially affected in ICC ( Supplementary Data 7 ). Although KRAS is the most frequently mutated gene (16.7%) in the Ras/PI3K signalling pathway, the alteration of this pathway is attributed also to many other genes including PTEN (5.9%), PIK3CA (3.9%), NF1 (3.9%) and EGFR (2.0%) known to be associated with many cancer types ( Fig. 4a ). Altogether, 72 ICC patients have mutations in one or more components of the Ras/PI3K signalling pathway ( P =1 × 10 −75 , Supplementary Data 6 ). Among the genes in the Ras/PI3K signalling pathway are cell membrane receptors, the ephrin receptors encoded by EPH genes including the significantly mutated gene EPHA4 ( Fig. 4a ). Although the role of ephrin–Eph interaction in cancer development is still obscure, it has been demonstrated that Eph receptors triggered by ephrins regulate Ras family proteins [46] and express highly in tumour cells [47] . Mutations in collagen, which is a component of extracellular matrix, are also enriched in ICC genomes (16%). As reported in previous studies, the expression of collagen, which is upregulated by Ras GTPase and PI3K/Akt signalling [48] , is elevated in tumour cells and plays a role in tumour progression and metastasis [49] , [50] . It is also suggested that genetic changes of gene COL1A2 may influence HCC risk and is thus likely involved in the pathogenesis of HCC [51] . These findings indicate distinctly mutated genes and pathways in ICC genomes involved in tumour development and progression comparing with HCC. Ras/PI3K signalling pathway is also affected in HCC genomes [13] . However, the genes that are mutated and their frequencies are dramatically different from those mutated in ICC. The most mutated Ras/PI3K signalling pathway components are KRAS and PTEN in ICC, while the most mutated components is RPS6KA3 (9.6%) in HCC [13] . p53 is a key component of the p53/cell cycle pathway, which also includes RB1 (4.9%). Altogether, 45 ICC patients have mutations in one or more of the p53/cell cycle pathway genes ( P =4 × 10 −42 , Fig. 4b ; Supplementary Data 8 ). The p53/cell cycle signalling pathway is also mutated in HCC [13] . The most commonly mutated gene of the p53/cell cycle in both ICC and HCC is TP53 (ref. 13 ). The TGF-β/SMAD4 signalling pathway component SMAD4 is significantly mutated in ICC patients ( P =2 × 10 −8 , Fig. 4c ). Altogether, 17 ICC patients have mutations in this pathway. In contrast ( Supplementary Data 6 ), the TGF-β/SMAD4 signalling pathway is not affected in HCC. Altered epigenetic regulation Recent sequencing efforts have revealed genes involved in chromatin remodelling and epigenetic regulation in HCCs [13] , [14] and in CCAs [22] . We curated a list of genes that have been demonstrated to play a role in epigenetic regulation based on previous publications [52] , [53] , [54] ( Supplementary Data 7 ). Our results show that in 102 ICC genomes, 77 epigenetic genes mutated in 53 patients ( Fig. 4d ; Supplementary Data 6 ). These genes are involved in different steps in epigenetic regulation, including DNA methylation, histone modification and chromatin remodelling [54] , [55] , [56] , [57] , [58] . Among these genes, ARID1A encodes a component of SWI/SNF chromatin remodelling complex and is also frequently mutated in HCC. In addition, genes encoding histone methyltransferase such as KMT2A / MLL , KMT2B / MLL2 , KMT2D / MLL4 are also found mutated in eight ICC patients in this study, as reported in other cancer genome sequencing studies [12] , [19] , [54] , [59] . Among 102 ICC patients in our cohort, five (4.9%) harbours mutations in IDH1 , and all mutations cluster in a previously reported hotspot (codon 132). Such clustering enables early detection of IDH1 mutation in circulating tumour DNA as a way to screen for potential ICC tumours. In contrast to many previous studies [23] , [24] , [41] , mutations in IDH2 were not found in our cohort of ICC patients. Mutations in IDH1 and IDH2 have been found to cause a gain-of-function in the production of 2-hydroxyglutarate and to alter histone and DNA methylation [60] . Recently, a target sequencing of IDH1 and IDH2 in a cohort of 326 ICC patients discovered 10% of patients mutated in IDH1 (ref. 41 ), which is relatively higher than that found in our cohort of ICC patients. However, both rates are much lower than that (19%) reported recently for ICC patients treated in the United States of America [24] , suggesting a high variation of mutation prevalence of IDH1 in different cohorts of ICC patients. The functional implication of IDH1 and IDH2 mutations is also variable among different cohort of ICC patients. Although mutations in IDH1 and IDH2 were associated with longer overall survival in one cohort of ICC patients [41] , they were associated with worse survival in another cohort of ICC patients [24] . Thus, the prognostic impact of mutations in IDH1 needs to be assessed with even larger cohort size. Epigenetic regulation is also altered in HCC [13] , however, these two types of PLCs show clear differences in the types of mutated genes. Mitochondrial gene mutations and defective oxidative phosphorylation In addition to somatic mutations in tumour-suppressor genes and oncogenes that trigger uncontrolled cell growth, somatic mutations in mitochondrial genes have been proposed to fuel cell growth by switching energy production through oxidative phosphorylation to glycolysis, which is known as the Warburg effect [61] . Mitochondrial function have been identified in a large array of cancer types and different cancer types or developmental states undergo different bioenergetic alterations [62] . Recent whole-genome sequencing effort found bioenergetic alterations in oxidative phosphorylation favours glycolysis in tumorigenesis [63] . Such mutations in protein-coding genes in the mitochondria genome have also been identified in HCC patients [64] , but have never been reported in ICC patients. Through comparative analysis of tumour and matching control sample pairs from ICC patients, we found 58 somatic mutations in the mitochondrial genome ( Supplementary Data 8 ). The ratio of mutant to wild-type bases in our ICC tumour samples range from 10.3% to 88.6%, with 37.9% of them higher than 50% ( Supplementary Data 8 ). Considering the possible heterogeneity of the tumour samples, this high percentage suggests that the many mutations are approaching homoplasmy within cells. Interestingly, in contrast to germline mutation found in the mitochondrial genome, these somatic mutations have relatively high impact on protein-coding genes ( Fig. 5 ). These somatic mutations resulted in significant mutations in MT-ND4 (8.8%), MT-ND5 (8.8%), MT-CO1 (7.8%), MT-ND1 (3.9%), MT-ND6 (3.9%) and MT-CO3 (3.9%), all of which encode proteins essential for the oxidative phosphorylation pathway. 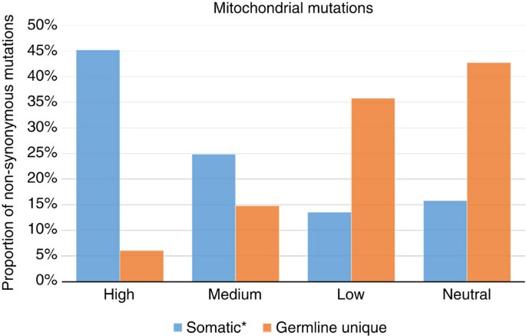Figure 5: Relative impact of somatic and germline non-synonymous mutations in ICC patients. Mutation impact was examined using MutationAssessor. Figure 5: Relative impact of somatic and germline non-synonymous mutations in ICC patients. Mutation impact was examined using MutationAssessor. Full size image To our best knowledge, this project is the first large-scale whole-exome sequencing project targeting ICC patients in China, and the cohort of ICC patients included in the discovery screen (102 patients) project is the largest among all such projects on ICC patients worldwide [22] , [23] , [24] . The scale of this project enabled us to uncover not only mutation spectrum shared by other cancer types, but also an ICC-unique mutation spectrum. The ICC-unique mutation spectrum (CTG>CAG and CAG>CTG) is tightly associated with liver inflammation, fibrosis and cirrhosis, suggesting that mutagens that have caused such mutations have also caused inflammation, fibrosis and cirrhosis. It is also likely that these ICC patients who harbour the ICC-unique mutation spectrum may have been exposed to aristolochic acid (AA), a nitrophenanthrene carboxylic acid found in all members of the genus Aristolochia plants that have been used in medicine for over 2,000 years [65] , [66] . Recent studies showed that humans exposed to AA causes A:T>T:A transversions [65] , [66] . AA has been demonstrated to be a causative carcinogen of urothelial carcinoma of the upper urinary tract (UTUC) [30] , [31] . Furthermore, A>T mutation rate observed in our ICC patients is comparatively higher on the non-transcribed strand ( Fig. 1e ), which is the same to that observed in AA-UTUC [30] , [31] . Further analysis of mutation signatures in TP53 revealed that aflatoxin is likely a risk factor for ICC in China. The large cohort size of ICC patients in this study also enabled us to identify 25 significantly mutated genes, including both genes previously known to be associated with ICC ( TP53 , KRAS , IDH1 , SMAD4 , AR1D1A and RB1 ) and novel genes ( PTEN , GOLGA6L2 , EPHA4 , EPPK1 , CDH18 , ALB , FAM182B, ECE2 , TDRD1 , GRIA1 , CNTNAP5 and FYN ) that have never been directly associated with ICC in previous studies. Our study further highlights that features of ICC: the genetic heterogeneity and the genetic uniqueness of different ICC cohorts. Combined mutation and clinicopathological analysis have showed that ICC patients who are positive for HBsAg are positively associated with the presence of mutations in TP53 , whereas those who are negative for HBsAg are positively associated with the presence of mutations in KRAS , suggesting different mechanisms in the tumorigenesis of ICC. HBsAg-seropositive ICC may share a common p53-mediated pathway with HBsAg-seropositive HCC [35] , thus usually show generally better prognosis compared with HBsAg-seronegative ICC [36] . Furthermore, HBsAg-seropositive ICC patients show different survival rates depending on the status of mutations in TP53 : HBsAg-seropositive ICC patients without mutations in TP53 have better survival than those with mutations in TP53 , suggesting that HBsAg-seropositive ICC patients may develop cancer through the interplay of multiple parallel mechanisms. In contrast, KRAS mutations are associated with worse prognosis, which may contribute to the overall worse survival of HBsAg-seronegative ICC patients. The uncovering of significantly mutated genes and pathways sets up a platform for further detailed molecular study of their contribution to ICC tumorigenesis. In particular, the uncovering of six mitochondrial genes that function in the oxidative phosphorylation in this whole-exome sequencing of ICC tumour and matching control samples underscores the importance of the mitochondrial genome in ICC tumorigenesis. This observation suggests that the Warburg effect [61] may exist in ICC and it may play an important role in ICC tumorigenesis. Results from this study also have potential profound impact on further clinical research and practice. Mutations, especially those that are found in the most commonly mutated genes including TP53 and KRAS may help us perform early diagnosis by detecting them using circulating cell-free DNA in the blood samples [67] . More importantly, significantly mutated genes identified in this study can all help develop targeted personalized therapies depending on the mutation landscape uncovered in each individual. Surgery All patients underwent anatomical en bloc resections, which resulted in partial hepatectomy (segmentectomy or bisegmentectomy or trisegmentectomy) in 84 patients (81.6%), a left hepatectomy in 13 patients (12.6%) and a right hemihepatectomy in 6 patients (5.8%). Concomitant caudate segmentectomy was carried out in two patients. Seven patients received common bile duct exploration for cholelithiasis or thrombus resection, and one patient received Roux-en-Y cholangiojejunostomy. If the tumour appeared to be invading adjacent organs grossly in the operative field, combined resection was performed to achieve complete removal of the tumour. An additional 49 combined resections of other organs were captured in 47 patients (45.6%). Among all patients, only one had surgical complication (biliary leakage). Specimen collection Tumour specimens were obtained from the tumour tissue and matched normal specimens were cut at the resection marge in which it is at least 3 cm from the tumour. The specimens were immediately frozen in liquid nitrogen and stored at −80 °C until DNA extraction. The investigation was approved by the Eastern Hepatobiliary Surgery Hospital Ethics Committee (Shanghai, China). Informed consent forms were signed before surgery. Statistical analysis Patients were screened for carcinoembryonic antigen, CA 19-9, and computed tomography scan every 1–2 months for the first 6 months after operation and every 3 months afterwards. When recurrence was suspected, magnetic resonance imaging or positron-emission tomography images were taken for confirmation. Disease-free survival was measured from the date of surgery to the date of recurrence. Survival was measured from the date of surgery. Follow-up of patients was continued until death or 7 July 2013. Statistical analyses were performed using SPSS, version 16.0 for Windows (SPSS Inc.). Comparisons between groups were conducted using the χ 2 test for categorical variables and the t -test for discrete variables. A value of P <0.05 was considered statistically significant. Whole-exome sequencing The 206 tumour/control paired samples isolated from 103 ICC patients were sequenced using commercial DNA sequencing services (WuXi AppTec, http://www.wuxiapptec.com/ ). Exome capturing was performed using NimbleGen SeqCap EZ Human Exome Library v3.0. Capture genomic DNAs were sequenced using Illumina HiSeq2000. Details of the exome sequencing results are summarized in Supplementary Data 2 . Exome sequencing results have been submitted to Short Read Archive database. Somatic point mutations and short indel calls Somatic point mutations and short indels were called in a procedure composed of five stages. First, the sequencing quality was examined by FastQC ( http://www.bioinformatics.babraham.ac.uk/projects/fastqc/ ). Second, the paired-end short reads were aligned to the Genome Reference Consortium human genome ( GRCh37 ) with default settings of Novoalign ( http://www.novocraft.com/main/index.php ). In this stage, reads with multiple alignments were discarded. Third, after sorting and removing PCR duplicates by SAMtools ( http://samtools.sourceforge.net/ ), variant identification was performed with VarScan2 ( http://varscan.sourceforge.net/ ). Fourth, we used PERL programming to identify somatic mutations with the following parameters: (i) base quality ≥20 (Fred quality score); (ii) read depth ≥15 in both tumour and control; (iii) Reads supporting variation ≥ (two in each strand) in tumour; (iv) variant allele frequency ≥10% in tumour; (v) reads supporting variation ≤2 in normal; (vi) NOT in dbSNP (Version 68, 2012-07-14) ( http://www.ncbi.nlm.nih.gov/SNP/ ) and the 1000 Genomes Project (Release v3, 2011-05-21) ( http://www.1000genomes.org/ ) unless the mutation is included in COSMIC database (Version 61, 2012-09-26) ( http://www.sanger.ac.uk/genetics/CGP/cosmic/ ). Fifth, all the somatic mutations were examined on GBrowse ( http://gmod.org/wiki/GBrowse ) and the impacts on protein sequences were annotated with CooVar [68] . Mutation validation by Sanger sequencing Genomic DNA of cancer and matched normal samples were used as PCR templates. PCR primers were designed for each somatic mutation using National Center for Biotechnology Information (NCBI) primer-BLAST ( http://www.ncbi.nlm.nih.gov/tools/primer-blast/ ). All primers designed and used in this project are listed in Supplementary Data 4 . Amplicons were then subjected to Sanger capillary sequencing (BGI). Amplicon sizes range from 200 to 1,600 bp. Each mutation was sequenced through both the forward and the backward directions. All sequencing results were aligned and visualized using chromas ( http://technelysium.com.au/ ). Identification of significantly mutated genes The significantly mutated genes are estimated by Genome-MuSiC [28] with default settings based on somatic mutations excluding those false positives by validation and those found in patient p119. The significant level is calculated in three statistical methods by Genome-MuSiC such as Fisher’s combined P -value test, Likelihood ratio test and Convolution test. Genes estimated significant by all of these three methods ( P <=0.05) were considered as significantly mutated genes (highlighted by light brown in Fig. 3 and in Supplementary Data 6 ). Identification of significantly altered pathways The significantly altered pathways were identified by Genome-MuSiC [28] with default settings. Genes were categorized into pathways based on literatures and KEGG pathway database ( http://www.kegg.jp/kegg/pathway.html ). The pathway table was prepared from the output of Genome-MuSiC pathscan (ran with default parameters), using KEGG and NCI pathways. Genome-MuSiC pathscan tests for the enrichment of mutated genes in these pathways, taking the mutation frequency into account (that is, a pathway in which the same gene is mutated in multiple patients is assigned a lower P -value). All pathways were then clustered using hierarchical average linkage clustering. The clustering is based on the amount of mutated genes that are shared between pathways (Jaccard index was used as similarity measure). That way, highly similar pathways sharing the same mutated genes can be shown next to each other in the output list. Thus, the order in the list was defined by the order in which these pathways appeared in the hierarchical tree (column ‘order’, sorted ascending). The pathways were filtered by statistical significance, hiding pathways with a P -value<1 × 10 −10 . For easy inspection, P -value was colour-coded to highlight the most significantly enriched pathways, assigning darker colours to lower P -values in the following tranches: <1 × 10 −40 (darkest); 1 × 10 −40 to 1 × 10 −30 ; 1 × 10 −30 to 1 × 10 −20 ; 1e × 10 −20 to 1 × 10 −10 (lightest). Within the P -value filtered list, pathway groups were defined by more or less arbitrarily cutting the hierarchical tree at a certain heights, resulting in distinct clusters. Each distinct cluster is assigned a different group number (column ‘group’). The remaining columns are explained below: Samples_Affected: Number of samples that had at least one gene mutated in this pathway; Total_Variations: Number of times genes were mutated across all samples; the same mutated gene is counted multiple times if it is mutated in multiple samples; P .value: P -value; FDR: false discovery rate; essentially a P -value adjusted for multiple testing; NumGenes: Total number of genes mutated across all samples; other than for ‘Total_Variations’, here genes are not counted multiple times if they are mutated in several patients; Genes: gene symbols of all mutated genes in this pathway, sorted alphabetically. Identification of mutation signature The mutation spectrum in Fig. 1a is described by mutation rate per Mb per patient based on all somatic mutations in 102 ICC genomes (p119 is excluded) including those in dbSNP and 1000 Genomes project. This triple-nucleotide mutational context is examined in both non-transcribed strand and transcribed strand, and then summarized in both strands ( Fig. 1f ). Mutation spectra were also compared among those patients with different clinical features including cirrhosis and hepatitis. The mutation signature is predict by tool EMu [27] with default settings, which used the data of mutational context as input and the triple-nucleotide context in reference genome as background. Structural impact of somatic mutations in significantly mutated genes For each gene, the coordinates of conserved domain were obtained from NCBI. NCBI blastp was then used with default settings to search for orthologues of seven representative species including gorilla ( Gorilla gorilla gorilla ), mouse ( Mus musculus ), rat ( Rattus norvegicus ), cat ( Felis catus ), chicken ( Gallus gallus ), rainbow trout ( Icorynchus mykiss ) and the African clawed frog ( Xenopus laevis ). Protein sequences of the putative cancer gene in human and its orthologues in these seven species were aligned using ClustalW ( http://www.ebi.ac.uk/Tools/msa/clustalw2/ ). Mitochondrial mutation impact Impact of non-synonymous single-nucleotide variants were determined by MutationAssessor [69] categorized into ‘high’, ‘medium’, ‘low’ and ‘neutral’ impact. Nonsense mutations and indels are considered as high impact. How to cite this article: Zou, S. et al. Mutational landscape of intrahepatic cholangiocarcinoma. Nat. Commun. 5:5696 doi: 10.1038/ncomms6696 (2014). Accession codes : The patient exome sequence data have been deposited in GenBank/EMBL/DDBJ Short Read Archive (SRA) under the accession code SRP045202 .